Fractal design concepts for stretchable electronics Stretchable electronics provide a foundation for applications that exceed the scope of conventional wafer and circuit board technologies due to their unique capacity to integrate with soft materials and curvilinear surfaces. The range of possibilities is predicated on the development of device architectures that simultaneously offer advanced electronic function and compliant mechanics. Here we report that thin films of hard electronic materials patterned in deterministic fractal motifs and bonded to elastomers enable unusual mechanics with important implications in stretchable device design. In particular, we demonstrate the utility of Peano, Greek cross, Vicsek and other fractal constructs to yield space-filling structures of electronic materials, including monocrystalline silicon, for electrophysiological sensors, precision monitors and actuators, and radio frequency antennas. These devices support conformal mounting on the skin and have unique properties such as invisibility under magnetic resonance imaging. The results suggest that fractal-based layouts represent important strategies for hard-soft materials integration. The field of stretchable electronics is of growing interest [1] , [2] , motivated both by fundamental considerations in material science and by application spaces in areas such as biomedicine [3] , [4] , [5] , [6] . A core challenge is in achieving high-performance electronic functionality with systems that offer elastic, low modulus responses to large strain deformations. Two of the most successful approaches to this problem exploit advanced composites, in a generalized sense. The first involves dispersing conducting or semiconducting nanomaterials (that is, nanowires, nanotubes or graphene) into elastomeric matrices [7] , [8] , [9] , [10] , [11] . Here, three-dimensional (3D) structures, including distributed networks of contacts, form spontaneously, but with limited direct control over key variables other than the overall loading fraction. The second exploits alternative classes of composites, created deterministically by using thin layers of electronic materials lithographically defined into two dimensional (2D) filamentary mesh layouts [12] , [13] , [14] . Advantages of this approach include the ability to co-integrate multiple high-performance material platforms with high spatial resolution and engineering control, in ways that also allow proper electrical contacts, both internal and external to the system [15] . An essential aim of both 3D random and 2D deterministic composites in stretchable electronics is to combine high loading of a hard component, for use in active devices, with overall mechanics that is dominated by a soft matrix, for stretchable response. This goal is opposite to that associated with traditional composites engineering and therefore demands alternative approaches. Here, we show that concepts in fractal geometry, which are known to determine behaviours in traditional 3D networks [16] , [17] , [18] , [19] , [20] and which are pervasive in biological systems including the human body [21] , [22] , can be successfully exploited in 2D deterministic systems, with important functional consequences in advanced stretchable electronics. Fractal-based structures can be described by self-similarity: subdivision into small sections yields pieces with geometries that resemble the whole. Compared with previously explored networks of periodic serpentine shapes, fractal designs can be engineered to accommodate enhanced elastic strain along a selected dimension and to support biaxial, radial and other deformation modes. In addition, the choices of topologies span a rich range, from lines to loops, capable of tailoring to specific electronic applications through integration and interdigitation of multiple structures. 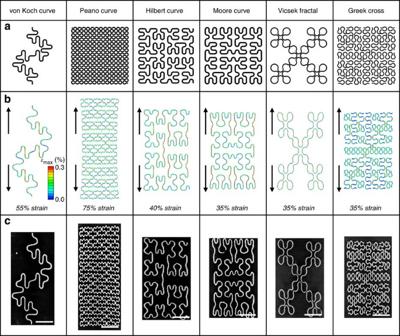Figure 1: Representative fractal-inspired layouts for hard-soft materials integration. (a) Six different patterns of metal wires fully bonded to elastomer substrates demonstrate the application of deterministic fractal designs as general layouts for stretchable electronics. These patterns include line, loop and branch-like geometries, and they are applicable to a broad range of active and passive electronic components. In all cases, arc sections replace the sharp corners from the mathematically defined fractal layouts to improve the elastic mechanics. (b) FEM images of each structure under elastic tensile strain and (c) their corresponding experimental MicroXCT images demonstrate the elastic mechanics. The wires consist of layers of gold (300 nm) sandwiched by polyimide (1.2 μm) and mounted on an elastomeric substrate (0.5 mm). Scale bars, 2 mm. Figure 1 presents six representative examples, from lines (Koch, Peano, Hilbert) to loops (Moore, Vicsek) and branch-like meshes (Greek cross). The results illustrate the diversity of possibilities, through both the finite element method (FEM) and experimental demonstration. The approximate fractal dimensions in these finite-iterative curves range from 1.5 to 2. The elastic tensile strains achieved with these structures indicate that they are suitable for use in various stretchable devices, including the epidermal electronic platform [23] , with key advantages over previously described layouts. Figure 1: Representative fractal-inspired layouts for hard-soft materials integration. ( a ) Six different patterns of metal wires fully bonded to elastomer substrates demonstrate the application of deterministic fractal designs as general layouts for stretchable electronics. These patterns include line, loop and branch-like geometries, and they are applicable to a broad range of active and passive electronic components. In all cases, arc sections replace the sharp corners from the mathematically defined fractal layouts to improve the elastic mechanics. ( b ) FEM images of each structure under elastic tensile strain and ( c ) their corresponding experimental MicroXCT images demonstrate the elastic mechanics. The wires consist of layers of gold (300 nm) sandwiched by polyimide (1.2 μm) and mounted on an elastomeric substrate (0.5 mm). Scale bars, 2 mm. Full size image Mechanics and electronics with Peano-based geometries The Peano curve [24] provides a model system for examining the detailed mechanics of fractal-based motifs. Layouts using these or other designs follow an iterative approach to create the Nth Peano curve, nine copies of the (N−1)th curve are linked together into a single line. An illustration of the first three iterations of a Peano curve appears in Fig. 2a . A physical interpretation that captures the underlying mechanics follows by considering the first iterative curve geometry as a section of a one-dimensional spring. Because of self-similarity, higher order Peano curves contain spring-like motifs at multiple length scales ( Supplementary Fig. 1 ). Furthermore, each of these motifs can be oriented vertically ( y -axis) or horizontally ( x -axis). As such, the Peano geometry provides a design metric for systematically ‘folding’ a straight line into a compact and stretchable layout. To further enhance the mechanics of these wires, arc sections replace the sharp corners in the mathematically defined Peano curves ( Fig. 2b ). Generally, the elastic mechanics of horseshoe serpentine structures improve with increasing arc section angle ( Supplementary Table 1 ). Although the Peano curves featured in Fig. 2a fill square areas, those of different iterative orders can be linked together to fill spaces of arbitrary shape. As a demonstration, Fig. 2c–f show the word ‘ILLINOIS’ formed with space filling wires, in which each letter consists of a combination of first and second order Peano curves. The figure includes a detailed view of a section of the ‘N’. Electrodes can be constructed in this manner to match, for example, particular features on the body. 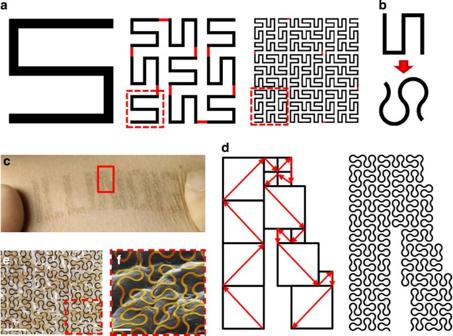Figure 2: Implementation of Peano curves for stretchable electronics. (a) Illustration of three iterations of a two-dimensional Peano curve. Nine versions of the (N-1)th curve (dotted red box) connect together with the solid red lines to construct the Nth curve. (b) Arc sections replace the sharp bends to enhance the mechanics. (c) Image of metal wires with Peano layouts, with an overall geometry that spell out the characters in ‘ILLINOIS’, mounted on skin. Here, each letter consists of a series of first and second order Peano curves. (d) A detailed section of the N (solid red box) from (c) in block diagram form (small blocks are first order curves, large blocks are second order curves) and as wires. (e) Optical and (f) scanning electron microscopy images of third order Peano-based wires on skin and a skin-replica (colorized metal wires), respectively, showing the conformal contact of the wires on the substrate. Scale bar in (e), 2 mm. Scale bar in (f), 500 μm. Figure 2: Implementation of Peano curves for stretchable electronics. ( a ) Illustration of three iterations of a two-dimensional Peano curve. Nine versions of the (N-1)th curve (dotted red box) connect together with the solid red lines to construct the Nth curve. ( b ) Arc sections replace the sharp bends to enhance the mechanics. ( c ) Image of metal wires with Peano layouts, with an overall geometry that spell out the characters in ‘ILLINOIS’, mounted on skin. Here, each letter consists of a series of first and second order Peano curves. ( d ) A detailed section of the N (solid red box) from ( c ) in block diagram form (small blocks are first order curves, large blocks are second order curves) and as wires. ( e ) Optical and ( f ) scanning electron microscopy images of third order Peano-based wires on skin and a skin-replica (colorized metal wires), respectively, showing the conformal contact of the wires on the substrate. Scale bar in ( e ), 2 mm. Scale bar in ( f ), 500 μm. Full size image The Peano curves in Fig. 2a represent only one set of variations; there exist many others, because the (N−1)th unit cells of any Nth order curve can be oriented either vertically or horizontally ( Supplementary Fig. 2 ). The second order curve has 272 unique layouts alone, each with distinct mechanical properties. Numerical simulations of five different second order layouts consisting of gold wires bonded on an elastomer probe the relationship between mechanics and layout. The layouts contain unit cells with orientations ranging from all vertical to all horizontal ( Table 1 ). The maximum principal strain criterion defines the maximum elastic stretchability as the onset of plastic yield, consistent with established parameters of the constituent materials [25] . Table 1 summarizes this quantity, calculated for uniaxial deformation along the x - and y -axis. The results indicate that Peano layouts with unit cells all oriented in the same way maximize the uniaxial stretchability along the unit cell direction. The ‘half-and-half’ Peano layout, which contains unit cells with alternating orientations, balances the maximum strain supported along the x - and y -axis at 16% and 13%, respectively. Such properties are well suited for devices that stretch along both axes. Adjustments to the total unit cell size can enhance the mechanics of these structures ( Supplementary Table 2 ). The third order half-and-half layouts yield stretchabilities along the x - and y -axis of 32% and 28%, respectively ( Supplementary Fig. 3 ). This improvement with iteration order is due to the combined effects of geometric scaling of the arc sections, increase in the length of the wire and addition of higher order spring-like motifs. The stretchability here is well above 20%, which is the general upper limit for the elastic mechanics of skin [23] . Table 1 Elastic mechanics of five different Peano-based wire structures. Full size table Experimental structures consisting of second and third order half-and-half Peano layouts of metallic wires that are clad with polyimide and fully bonded to an elastomeric membrane compare well with the numerical analysis (See Methods for details). The polyimide cladding retards strain localization in the metal [26] , thereby enhancing sample yield and consistency in the mechanical tests. Three samples are tested for each fractal dimension and axis of stretching. Mechanical characterization involves measurements of resistance changes to a precision of ~0.01 ohms with a four-point probe technique performed during uniaxial tensile stretching. In the elastic regime, the wire resistance before and after cycling between states of no strain and increasing levels of maximum strain (the difference defined as the ‘differential resistance’) does not change. At the onset of plastic deformation, the wire undergoes a resistance-dependent geometric change, leading to a small but measurable differential resistance. Traditional approaches to characterizing plasticity [27] , [28] based on measurements of stress-strain response with a tensometer are not suitable because the mechanics of the elastomeric substrates in these systems dominate the response, by design. 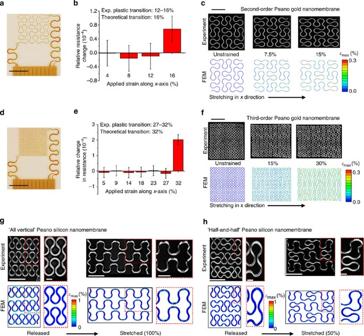Figure 3: Mechanics of metal and semiconductor fractal-based structures. (a,d) Optical images of metal wires patterned with second and third order half-and-half Peano layouts. The samples connect to a stretchable set of four wires used for four-point probing. Scale bar, 5 mm. (b,e) Plot of differential resistances measured at increasing levels of maximum applied strain. The onset of plastic deformation corresponds to the strain at which the differential resistance is non-zero. (c,f) A comparison between experimental optical images and FEM-constructed images of the second and third order structures for different levels of stretching. The FEM images display localized areas of high strain in the stretched structures. Scale bar, 3 mm. (g,h) MicroXCT and FEM images of Si NMs patterned into Peano layouts and fully bonded to a 40% pre-strained elastomeric substrate. Upon release and uniaxial stretching, both structures dissipate the mechanical stress via microscale buckles, which is indicative of a mechanical regime well suited for high levels of elastic deformation. Scale bar, 1 mm. Figure 3a–f and Supplementary Fig. 3 summarize the results of these studies. The differential resistances measured from individual representative devices appear together in each plot. The error bars in the second and third order Peano structures have magnitudes of 3.7e-5 and 3.3e-5, respectively; Supplementary Note 3 discusses the sources of these errors. Simultaneous measurements of the local temperature account for and calibrate out changes in resistance due to background temperature fluctuations (See Supplementary Note 2 ). The measurements show that for the second order Peano structures stretched along the x - and y -axis, the transition from elastic to plastic deformation occurs in the range of 16–20% and 12–16%, respectively. The third order Peano structures undergo an elastic-to-plastic transition in the range of 27–32% for stretching along both x - and y -axes. These values of uniaxial stretchability are consistent with the numerical analysis. Calculated FEM images of strain localized in the stretched structures ( Fig. 3c,d ) display the positions of the mechanical ‘hot spots’ in the samples, where strains are particularly large and where failure occurs. Further enhancements in device mechanics are possible by optimizing the detailed geometry of these hot spots. Figure 3: Mechanics of metal and semiconductor fractal-based structures. ( a , d ) Optical images of metal wires patterned with second and third order half-and-half Peano layouts. The samples connect to a stretchable set of four wires used for four-point probing. Scale bar, 5 mm. ( b , e ) Plot of differential resistances measured at increasing levels of maximum applied strain. The onset of plastic deformation corresponds to the strain at which the differential resistance is non-zero. ( c , f ) A comparison between experimental optical images and FEM-constructed images of the second and third order structures for different levels of stretching. The FEM images display localized areas of high strain in the stretched structures. Scale bar, 3 mm. ( g , h ) MicroXCT and FEM images of Si NMs patterned into Peano layouts and fully bonded to a 40% pre-strained elastomeric substrate. Upon release and uniaxial stretching, both structures dissipate the mechanical stress via microscale buckles, which is indicative of a mechanical regime well suited for high levels of elastic deformation. Scale bar, 1 mm. Full size image Fractal-based structures bonded to pre-strained elastomers enable higher levels of elastic deformation [29] , [30] . A second order all-vertical Peano structure fully bonded onto an elastomeric substrate with 40% pre-strain demonstrates the concept. The differential resistances for different levels of maximum applied strain appear in Supplementary Fig. 4 . Here, the transition from elastic to plastic deformation occurs when the substrate is strained in the range of 60–70%, which is significantly higher than that in samples prepared without pre-strain. Schemes that use pre-strain can be extended to biaxial, radial or other types of deformation. This concept of enhancing mechanics through the use of pre-strain is general to a broad range of materials, including semiconductors. Thin films of single crystalline silicon nanomembranes (Si NM) with two different second order Peano layouts and bonded onto 40% pre-strained elastomeric substrates provide a proof of concept. In the pre-strained state, the calculated compressive stresses in the membrane are well within the regime of elastic deformation for silicon. Figure 3g,h shows microscale X-ray coherent tomography (microXCT, see Supplementary Note 1 ) images of the samples, along with corresponding FEM results. The findings indicate that the all-vertical and half-and-half structures can be elastically strained by 105% and 63%, respectively, given a maximum principal strain of 1% in the silicon [31] . The fracture points measured electrically from half-and-half structures ( Supplementary Fig. 5 ) are consistent with the FEM results. Both the microXCT and FEM images reveal microscale buckling; this type of deformation mode improves the ability of the Si NMs to dissipate stress. Such behaviour persists only for a limited range of NM thicknesses. FEM simulations show that, with increasing membrane thickness, the NMs transition from a regime of wrinkling to microscale buckling and finally to global buckling; furthermore, the microscale buckling regime yields maximal elastic mechanics ( Supplementary Fig. 6 ). As such, the optimization of the elastic properties of hard-soft systems requires careful attention to micro-mechanics. Fractal-based epidermal electronics The Peano and other fractal layouts have utility for various applications. One is in skin-mounted sensors and actuators such as temperature sensors, heaters and electrodes ( Supplementary Fig. 7 ). Electrodes measure electrophysiological processes in the brain (electroencephalograms (EEGs)) [23] , heart (electrocardiograms (ECGs)) and muscle (electromyograms (EMGs)) [32] , [33] . To minimize impedance between the electrode and skin and to optimize the measured signal-to-noise, electrodes require both conformal skin contact and high areal coverage [32] , [33] . Electrodes that interface directly with neurons additionally benefit from having large perimeters within an area [34] , [35] , [36] . These needs can be addressed effectively using a variant of the Greek cross fractal, which consists of a hierarchy of cross structures that fills space in two dimensions ( Supplementary Fig. 8 ). This design embeds a high level of connectivity, which minimizes the resistance between any two points. In addition, defects in the structure, such as line breaks, have a reduced probability for significantly affecting device performance, which is desirable for robust, long-term health monitoring in practice [33] . These geometries can be further designed to eliminate closed loops ( Supplementary Fig. 8 ), such that the edges of the electrode wire layout form a single continuous line. A multifunctional device that incorporates a resistive temperature sensing/heating element with an integrated electrode (recording, ground and reference components together) exploits this feature [30] ( Fig. 4a ). The temperature sensor [37] consists of an insulated line of metal running along the edges of the Greek cross electrode. 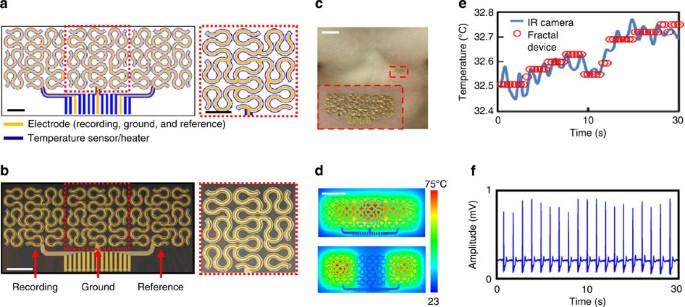Figure 4: Fractal-based epidermal devices. (a) Schematic image of a multifunctional device based on a Greek cross fractal design, with corresponding images of the device on a wafer (b) and mounted on skin (c). The device has multiple operation modes, including those for (d) Joule heating, by driving currents through the insulated heater wires, (e) temperature sensing via four-point probing, and (f) ECG measurements, in which the patch integrates the recording, reference and ground electrodes. Scale bars in (a) and (b), 2 mm. Scale bars in (c) and (d), 5 mm. Figure 4b–f shows a representative device and its operation under different modes (heating, temperature sensing, ECG measurements). The impedances and signal-to-noise measured with these dry electrodes compare favourably to that of conventional gel-based electrodes ( Supplementary Fig. 9 ), indicating that they are suitable for high quality, skin-mounted, electrophysiological measurements. The precision of the temperature measurement (~20 mK) compares well with that of an infrared camera. Figure 4: Fractal-based epidermal devices. ( a ) Schematic image of a multifunctional device based on a Greek cross fractal design, with corresponding images of the device on a wafer ( b ) and mounted on skin ( c ). The device has multiple operation modes, including those for ( d ) Joule heating, by driving currents through the insulated heater wires, ( e ) temperature sensing via four-point probing, and ( f ) ECG measurements, in which the patch integrates the recording, reference and ground electrodes. Scale bars in ( a ) and ( b ), 2 mm. Scale bars in ( c ) and ( d ), 5 mm. Full size image Radio-frequency devices with fractal layouts Stretchable radio frequency antennas, which are broadly applicable as mechanically-tunable electronic components [38] , [39] , are another class of devices that benefit from concepts in fractal design. Fractal antennas have been a topic of interest because they can support multiband operation in spatial scales that are compact relative to the resonant wavelength [40] , [41] , [42] . Appropriate choices of fractal layout offer not only this characteristic but also attractive elastic mechanics when mounted on stretchable substrates. A Vicsek curve loop antenna ( Supplementary Fig. 10 ), in which arc sections replace sharp bends, provides a model system. The antenna consists of copper traces (3 μm thick) laminated with polyimide, and bonded onto a 1 mm thick elastomeric substrate. The copper thickness is comparable to the skin depth of copper (~2 μm) at gigahertz frequencies. The return loss spectrum for the unstrained antenna displays a fundamental mode near 1.7 GHz ( Fig. 5a ) with an impedance of 42 ohms at resonance. The total length of the antenna at resonance is approximately λ 0 /6, where λ 0 is the free space wavelength, reflecting the compact nature of this particular fractal layout. As the device is strained, its fundamental frequency and input impedance slightly shift. Far-field measurements in an anechoic chamber provide additional information; data for the fundamental mode at 0 and 30% strain ( Fig. 5c ) display a clear dipole-like pattern. The realized gain for both the unstretched and stretched devices ranges from −2 to 0 dB, which is slightly less than that for an ideal dipole due to ohmic losses in the thin copper wires. Simulations of the return losses and far field profiles are consistent with the experiments ( Supplementary Fig. 11 , Supplementary Note 4 ). 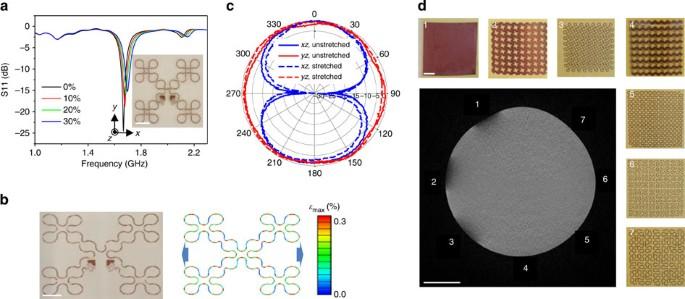Figure 5: RF properties of stretchable fractal structures. (a) Return loss parameters of a box fractal antenna under different amounts of tensile strain. Inset: optical image of an unstrained antenna fully bonded onto an elastomer. Scale bar, 4 mm. (b) Optical image of a box fractal antenna under 30% tensile strain and a corresponding FEM-constructed image of the same structure. Scale bar, 4 mm. (c) Far-field profiles of the antenna under no strain and 30% strain. (d) Cross-sectional MRI image of different copper samples (labelled 1-7) attached to a bottle of water. The solid and mesh samples display shadowing in the MRI image, while the fractal-based samples display no such shadowing. The sample layouts all are 1 × 1 inches and are (1) solid square, (2) thick mesh, (3) thin mesh, (4) horizontal and vertical stripes separated by a spacer, (5) Peano curve, (6) Hilbert curve, (7) Serpentine Greek cross. Scale bar, 5 mm. Figure 5: RF properties of stretchable fractal structures. ( a ) Return loss parameters of a box fractal antenna under different amounts of tensile strain. Inset: optical image of an unstrained antenna fully bonded onto an elastomer. Scale bar, 4 mm. ( b ) Optical image of a box fractal antenna under 30% tensile strain and a corresponding FEM-constructed image of the same structure. Scale bar, 4 mm. ( c ) Far-field profiles of the antenna under no strain and 30% strain. ( d ) Cross-sectional MRI image of different copper samples (labelled 1-7) attached to a bottle of water. The solid and mesh samples display shadowing in the MRI image, while the fractal-based samples display no such shadowing. The sample layouts all are 1 × 1 inches and are (1) solid square, (2) thick mesh, (3) thin mesh, (4) horizontal and vertical stripes separated by a spacer, (5) Peano curve, (6) Hilbert curve, (7) Serpentine Greek cross. Scale bar, 5 mm. Full size image Another application that can benefit from the favourable RF properties and mechanics of fractal patterns is in electrode structures that are compatible with magnetic resonance imaging (MRI). Copper foil samples mounted onto a cylindrical phantom and scanned in a 3-Tesla Trio head scanner (Siemens Instriuments) provide a demonstration. For purposes of comparison, the samples include three types of fractals, along with an unpatterned sheet, two variants of serpentine meshes, and superimposed vertical and horizontal lines. The fill fraction of the meshes and the fractal patterns are approximately the same (~25%). For the magnetic field strength used here, the resonant RF pulse frequencies are ~123 MHz. Figure 5d displays an axial cross-sectional scan obtained using a spin echo imaging sequence (parameters are in Supplementary Note 5 ). The water-based phantom appears white due to its high hydrogen concentration. The MRI image shows clear shadows in the vicinity of the unpatterned film and the mesh samples. Conversely, the fractal samples exhibit no noticeable distortion or shadowing. Magnetostatic coupling between RF radiation and the samples, which yields circulating currents and associated heat dissipation and signal loss, explains these differences. The meshes couple to RF radiation because they consist of highly interconnected closed loops of metal; in contrast, the fractals do not contain closed loops, do not couple to RF radiation and are invisible in the MRI. This analysis suggests that fractal-based designs provide routes to MRI-compatible skin-mounted or implanted electronic devices. In summary, fractal-based layouts create new design opportunities in stretchable electronics, including a broad range of devices suitable for biomedical systems. One of the challenges here is evaluating the mechanical properties of these composite materials and rigorously identifying their elastic and plastic mechanics. With the combination of high precision electro-mechanical measurements and three-dimensional FEM simulations, the fundamental mechanical responses and their dependence on geometry can be understood and exploited for specific deformation modes. This study suggests a general relationship between fractal layouts and mechanics that is broadly applicable to stretchable materials engineering. Epidermal device fabrication Fabrication of metal-based devices, including the temperature sensors and heaters, involves first spin-coating and curing liquid polyimide (PI) on a UV-treated PDMS-coated Si wafer. Electron beam evaporation yields layers of chromium (4 nm) and gold (300 nm). Following metal patterning, etching and the application of a second layer of polyimide, a photoresist mask and oxygen plasma etch define the polyimide-encapsulated device. All of the wires are 70 μm wide and the polyimide layers are each 1.2 μm thick. Water-soluble tape (3 M) retrieves the gold-polyimide structures, which covalently attach to an elastomer (0.5 mm thick, Ecoflex or Solaris, Smooth-on Inc.) using an evaporated chromium-silica bonding layer. UV radiation pretreatment of the elastomer promotes covalent bonding between the silica and elastomer. An ACF cable (Elform, USA) attached to the bonding pads of the device enable accessible electrical addressing. The same process, with an additional polyimide etch step, applies to the open metal-based fractal electrodes for electrophysiological sensing. An SOI wafer consisting of 260 nm thick p-doped silicon on a 1 μm thick silicon dioxide layer is the starting point for the Si NM samples. To detach the Si NMs from the handle wafer, an HF wet etch dissolves the underlying silicon dioxide through an array of 3 μm wide holes defined in the membranes. A PDMS stamp transfers the membranes onto a polyimide film, and a photoresist mask and dry etching process define the membranes into various Peano layouts. Gold wires electrically address the devices, and the same transfer steps described above finalize the devices. Antenna fabrication The starting material is copper foil (3 μm) on a copper carrier (35 μm; Olin Brass). Polyimide spun-cast and cured onto the foil yield foil-polyimide laminates, which mount onto a PDMS-coated substrate and enable copper carrier removal. A photoresist mask, wet copper etch and oxygen plasma dry etch pattern the antenna. Fractal-based metal wire simulations FEM yields the theoretical deformation, elastic-to-plastic transition and fracture of the structures. For simulations presented in Figs 1 and 3 and Table 1 , the elastomeric substrates employ an 8-node, hexahedral brick solid element C3D8R in the FEM programme, and the thin wires of PI/Au/PI-layered geometry employ a quadrilateral shell element S4R with the section of composite layup. All of the wires are 70 μm wide and consist of a 300 nm thick gold layer sandwiched by 1.2 μm thick polyimide layers on each side. The total pattern areas are 7 by 7 mm and fully bond to a 0.5 mm thick elastomer with a modulus of 50 kPa. The solid elements bond together physically and therefore share nodes with its adhered shell elements. An ideal elastic-plastic constitutive relation with a Young’s modulus of 78 GPa, Poisson’s ratio of 0.44, yield strain of 0.3% and fracture strain of 5% describe the mechanical behaviour of Au. The elastic-plastic transition is set when the maximum strain of half the width of one section is beyond the yield strain of 0.3%. Electrode and temperature sensor testing The Greek cross electrodes record ECG signals from the torso. Scotch tape exfoliates the stratum corneum and an alcohol swab removes dirt or particles to reduce effects of hydration and surface impedance. Here, the ground electrode, located between the measurement and reference electrodes (~7 mm apart at center-to-center distance), defines the common zero potential. Measured signals transmit wirelessly to a receiver, and commercial software using a 60 Hz notch filter and low-pass Butterworth filters (BioRadio 150, Cleveland Medical Devices, USA) completes the analysis. The fractal temperature sensors operate using the same four-point probe technique described in the mechanical testing section. An IR camera and hot plate yields d V/ d T used to calibrate the devices. The devices mount directly onto the skin with no elastomeric backing layer with a spray bandage technique. All experiments on human skins were conducted under approval from Institutional Review Board at the University of Illinois at Urbana-Champaign (protocol number: 13261). There are two subjects (age: 21~32, all males), co-authors in the paper. Research was carried out with informed signed consents from the subjects. How to cite this article: Fan, J. A. et al . Fractal design concepts for stretchable electronics. Nat. Commun. 5:3266 doi: 10.1038/ncomms4266 (2014).